Three-dimensional orientation-unlimited polarization encryption by a single optically configured vectorial beam The interplay between light polarization and matter is the basis of many fundamental physical processes and applications. However, the electromagnetic wave nature of light in free space sets a fundamental limit on the three-dimensional polarization orientation of a light beam. Although a high numerical aperture objective can be used to bend the wavefront of a radially polarized beam to generate the longitudinal polarization state in the focal volume, the arbitrary three-dimensional polarization orientation of a beam has not been achieved yet. Here we present a novel technique for generating arbitrary three-dimensional polarization orientation by a single optically configured vectorial beam. As a consequence, by applying this technique to gold nanorods, orientation-unlimited polarization encryption with ultra-security is demonstrated. These results represent a new landmark of the orientation-unlimited three-dimensional polarization control of the light–matter interaction. Control of the light polarization state is fundamental to the light-matter interaction in a variety of applications, including polarization information encryption [1] , [2] , multi-dimensional optical data storage [3] , nonlinear optics [4] , imaging [5] , [6] and surface plasmon-based photonic devices [7] , [8] . Creating an arbitrary three dimensional (3D) light polarization orientation has never been achieved, although it is essential to the interaction between light and 3D physically anisotropic micro- and nano-objects [9] , [10] , [11] . The electromagnetic wave nature of light in free space confines the polarization orientation control only to planar regimes. A way to break this limit is to bend the wavefront of light through vectorial diffraction by a high numerical aperture (NA) objective lens [12] , [13] . Although a longitudinal polarization state can be created by focussing a radially polarized light beam [14] , [15] , [16] , there has been a key obstacle of generating arbitrary 3D polarization orientation in the focus. Here we demonstrate a breakthrough of 3D arbitrary polarization orientation control using single optically configured vectorial beams. The optical configuration of a single vectorial beam is based on the superposition of a radially polarized beam and an azimuthally polarized beam. The vectorial diffraction of the superposed beam by a high NA objective lens can construct arbitrary 3D polarization orientation. This kind of focal polarization control enables us to achieve an orientation-unlimited polarization information encryption when it is applied to gold nanorods. Consequently, the 3D arbitrary 'key' polarization generation capability facilitates the polarization encryption with ultra-security. Arbitrary 3D polarization orientation The key to achieving arbitrary 3D polarization orientation control is to superpose a radially polarized beam and an azimuthally polarized beam with weighting factors γ and δ , respectively, as illustrated in Fig. 1a . Then, the amplitude of the single vectorial beam is modulated by an apodizer with a pupil function P ( α , ), where α and is the azimuthal angle of the transmission apertures and the normalized radius of the obstruction within an apodizer, respectively ( Supplementary Fig. S1 ). At the input plane of the objective lens, the single vectorial beam can be written as E = P ( α , )( γ · e r + δ · e φ ), where e r and e φ are the unit vectors in the radial and azimuthal directions, respectively. 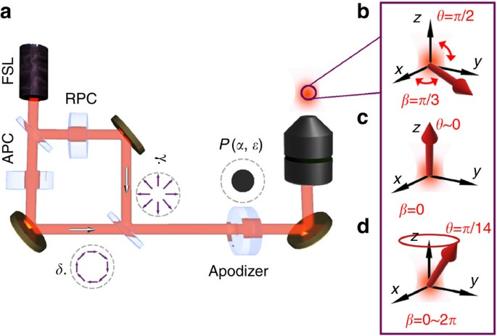Figure 1: Arbitrary 3D polarization orientation achieved by a single optically configured vectorial beam. (a) Schematic illustration of the parametric configuration of a single vectorial beam. FSL represents femtosecond laser. APC and RPC represent azimuthal and radial polarization convertors, respectively.γandδare weighting factors of radially and azimuthally polarized beams, respectively.P(α,) is the pupil function of the apodizer, whereαandare the azimuthal angle of the transmission apertures and the normalized radius of the obstruction within the apodizer, respectively. (b–d) Examples of resultant 3D polarization with (b) in-plane orientation (θ=π/2,β=π/3) configured at γ=0,δ=1 and P(α= 5π/6,=0), (c) out-of-plane orientation (θ~0,β=0) configured atγ=1,δ=0 andP(α=0,=0.7), and (d) 3D orientation (θ=π/14,β= 0 ~ 2π) configured atγ=1,δ=0 andP(α=0,=0). Figure 1: Arbitrary 3D polarization orientation achieved by a single optically configured vectorial beam. ( a ) Schematic illustration of the parametric configuration of a single vectorial beam. FSL represents femtosecond laser. APC and RPC represent azimuthal and radial polarization convertors, respectively. γ and δ are weighting factors of radially and azimuthally polarized beams, respectively. P ( α , ) is the pupil function of the apodizer, where α and are the azimuthal angle of the transmission apertures and the normalized radius of the obstruction within the apodizer, respectively. ( b – d ) Examples of resultant 3D polarization with ( b ) in-plane orientation ( θ = π /2, β = π /3) configured at γ=0, δ =1 and P( α = 5 π /6, =0), ( c ) out-of-plane orientation ( θ ~0, β =0) configured at γ =1, δ =0 and P ( α =0, =0.7), and ( d ) 3D orientation ( θ = π /14, β = 0 ~ 2 π ) configured at γ =1, δ =0 and P ( α =0, =0). Full size image By configuring the three parameters ( γ , δ , P ) of the single vectorial beams, the ratio of the averaged longitudinal polarization component ( I z ) to the averaged transverse polarization component ( I p ) within the focal plane defined by the full-width at half-maximum (FWHM) can be freely tunable to construct arbitrary 3D polarization orientation in the focus of the objective (see Methods ). Depending on the parametric configuration, the resultant polarization orientation can be within the focal plane (in-plane: θ = π /2, β = π /3), perpendicular to the focal plane (out-of-plane: θ ~0, β =0) or in an arbitrary direction ( θ = π /14, β = 0 ~ 2 π ), as exemplified in Fig. 1b–d , respectively, where θ is the out-of-plane angle with respect to the z axis and β is the in-plane angle with respect to the x axis. Most importantly, the judicious parametric configuration of the single vectorial beam enables both out-of-plane and in-plane orientation angles to be continuously adjustable, therefore giving rise to an orientation-unlimited flexibility of controlling the focal polarization direction ( Supplementary Fig. S2 ). In contrast to the recent analytical proposals for 3D polarization control [17] , [18] , our method shows the 3D orientation-unlimited flexibility as well as the simple input polarization configuration. As a demonstration of the arbitrary 3D polarization orientation control, we apply the single optically configured vectorial beam to excite gold nanorods, which have an anisotropic polarizability. When the configured beam polarization interacts with randomly aligned nanorods, it can selectively excite those nanorods aligned parallel with the polarization direction, as illustrated in Fig. 2a . Therefore, illumination by a given configured vectorial beam enables the determination of the alignment angles ( θ , β ) of gold nanorods in single raster scanning fluorescence images. To this end, we calculated the two-photon fluorescence (TPF) rate image [19] of gold nanorods with different alignment angles (see Methods ) for a single vectorial beam configured with the parameters of γ =1, δ =0 and P ( α =0, =0.7). The gold nanorods with in-plane, out-of-plane, and arbitrary 3D alignments can be clearly distinguished by their intensity patterns in the fluorescence scanning images, as shown in Fig. 2b–e . The TPF imaging experiment of gold nanorods [6] was performed in a homebuilt microscope (see Methods ). 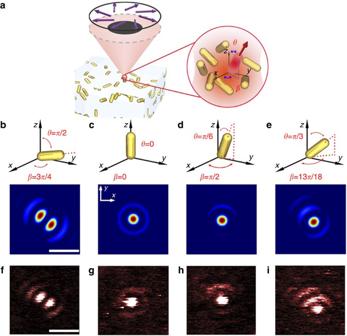Figure 2: Three-dimensional alignment determination of single gold nanorods in TPF scanning images. (a) Schematic illustration of an arbitrary 3D polarization beam interacting with randomly aligned gold nanorods with out-of-plane angleθand in-plane angleβ. The purple arrows and the black circle represent the input polarization state of the single vectorial beam and the back aperture of the objective, respectively. The dashed circle and black disc represent the apodizer. The focal polarization is indicated by the red arrow. (b–e) Schematic 3D alignment of gold nanorods and their associated calculated fluorescence rate images. (f–i) Experimental results of TPF images of gold nanorods with the corresponding orientation. (b) and (f), a nanorod aligned atθ=π/2,β= 3π/4; (c) and (g), a nanorod aligned atθ=0,β=0; (d) and (h), a nanorod aligned atθ=π/6,β=π/2; (e) and (i), a nanorod aligned atθ=π/3,β= 13π/18. Scale bar, 1 μm. Figure 2f–i is the experimental result of TPF scanning images of single gold nanorods with different alignment angles, which are in perfect agreement with the calculations. Scanning electron microscope images of corresponding gold nanorods ( Supplementary Fig. S3 ) were obtained to confirm the alignment angles measured in the TPF experiment in a reasonable accuracy ( Supplementary Table S1 and Supplementary Discussion ). Figure 2: Three-dimensional alignment determination of single gold nanorods in TPF scanning images. ( a ) Schematic illustration of an arbitrary 3D polarization beam interacting with randomly aligned gold nanorods with out-of-plane angle θ and in-plane angle β . The purple arrows and the black circle represent the input polarization state of the single vectorial beam and the back aperture of the objective, respectively. The dashed circle and black disc represent the apodizer. The focal polarization is indicated by the red arrow. ( b – e ) Schematic 3D alignment of gold nanorods and their associated calculated fluorescence rate images. ( f – i ) Experimental results of TPF images of gold nanorods with the corresponding orientation. ( b ) and ( f ), a nanorod aligned at θ = π /2, β = 3 π /4; ( c ) and ( g ), a nanorod aligned at θ =0, β =0; ( d ) and ( h ), a nanorod aligned at θ = π /6, β = π /2; ( e ) and ( i ), a nanorod aligned at θ = π /3, β = 13 π /18. Scale bar, 1 μm. Full size image Orientation-unlimited selective excitation of gold nanorods The capability of generating arbitrary 3D polarization orientation allows us to achieve the orientation-unlimited selective melting of the gold nanorods provided that the excitation beam power exceeds the threshold [20] . To characterize the melting rate under the illumination of a single optically configured vectorial beam, we studied the TPF contrast reduction (see Methods ) of gold nanorods. 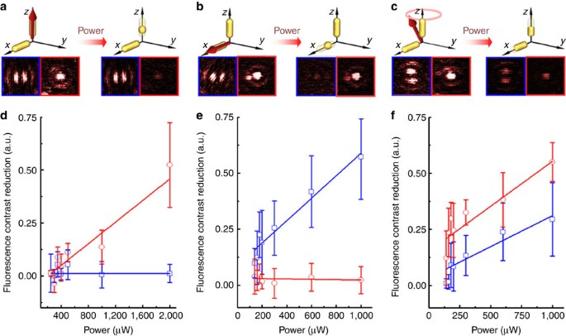Figure 3: Orientation-unlimited selective excitation and melting of gold nanorods. The fluorescence contrast reduction for the excitation and melting of nanorods under the illumination of the three differently oriented polarization beams configured at (a)γ=1,δ=0 andP(α=0,=0.7); (b)γ=0, δ=1 and P(α=π/2,=0); (c)γ=1,δ=0 and P(α=0,=0). The measurements are averaged over 15 gold nanorods. The experimental results of nanorods with in-plane and out-of-plane alignments are denoted by blue and red colours, respectively. (a–c) The schematic illustration of the gold nanorod alignment with respect to the three polarization orientations, indicated by the red arrows, and the corresponding TPF images of the given nanorods with in-plane (blue border) and out-of-plane (red border) alignments, before and after exposure to the three polarization orientations. (d–f) The fluorescence contrast reduction as a function of the illumination power. The error bars reflect s.d. The linear fits are a guide for the eye. Figure 3a–c shows the scheme of the photothermal reshaping of nanorods and the TPF images of two nanorods with in-plane (blue) and out-of-plane (red) alignments, respectively, before and after melting, when exposed to three polarization orientations of the single configured vectorial beam. Figure 3: Orientation-unlimited selective excitation and melting of gold nanorods. The fluorescence contrast reduction for the excitation and melting of nanorods under the illumination of the three differently oriented polarization beams configured at ( a ) γ =1, δ =0 and P ( α =0, =0.7); ( b ) γ =0, δ=1 and P( α = π /2, =0); ( c ) γ =1, δ =0 and P( α =0, =0). The measurements are averaged over 15 gold nanorods. The experimental results of nanorods with in-plane and out-of-plane alignments are denoted by blue and red colours, respectively. ( a – c ) The schematic illustration of the gold nanorod alignment with respect to the three polarization orientations, indicated by the red arrows, and the corresponding TPF images of the given nanorods with in-plane (blue border) and out-of-plane (red border) alignments, before and after exposure to the three polarization orientations. ( d – f ) The fluorescence contrast reduction as a function of the illumination power. The error bars reflect s.d. The linear fits are a guide for the eye. Full size image Figure 3d–f shows the averaged TPF reduction as a function of the illumination power. As shown in Fig. 3d , when a longitudinal polarization state ( θ ~0) of the single vectorial beam is used, the gold nanorods with the out-of-plane alignment can be melted quickly whereas those with the in-plane alignment remain unaffected, where the transverse polarization intensity component contributes less than 5% of the total energy within the FWHM-defined focal plane. A reversed situation is observed when the polarization of the single vectorial beam is configured to be in-plane ( Fig. 3e ). Finally, Fig. 3f shows the nearly identical melting rates in out-of-plane- and in-plane-aligned gold nanorods when excited by the polarization beam with θ = π /14. These features clearly demonstrate the orientation-unlimited flexibility of selective melting when a single vectorial beam is optically configured by the three parameters. 3D orientation-unlimited polarization encryption This orientation-unlimited property gives rise to the ultra-security polarization information encryption for a given region. Using this technique, we demonstrate the 3D five-state polarization encryption. To prevent the unselected gold nanorods from the influence of the accumulative temperature rise of the polymer matrix [21] , [22] , the pulse repetition rate was optimized at 1 kHz (see Methods and Supplementary Fig. S4 ). The laser power used for encryption was optimized to minimize the cross-talk ( Supplementary Fig. S5 and Supplementary Discussion ) between different polarization orientations. In Fig. 4a–e , we show five TPF raster scanning images encrypted at the same region by the five configured polarization orientations of the single vectorial beam indicated by the direction of red arrows. Each pattern consisting of 75 by 75 pixels, with a pixel separation of 0.55 μm, was encrypted in a homebuilt confocal microscope (see Methods ). The exposure time for each pixel was 30 ms. The encrypted information was retrieved by TPF imaging through raster scanning at a reduced power level. The encrypted information can only be retrieved when read by the 'key' polarization orientation, which is the same as that during the encryption, otherwise the information is read out as noise. These results indicate that polarization information encryption with an orientation-unlimited flexibility, and ultra-security is feasible using the demonstrated technique. 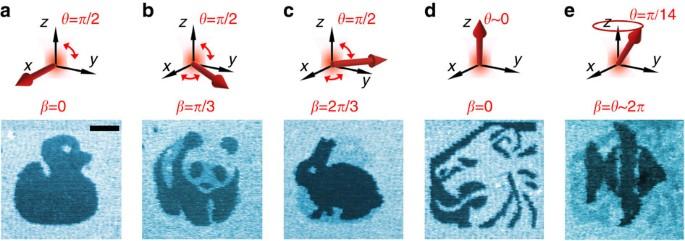Figure 4: Demonstration of 3D orientation-unlimited polarization encryption. The red arrows in (a–e) indicate the five configured polarization orientations used for the information encryption at (a)θ=π/2,β= 0, (b)θ=π/2,β=π/3, (c)θ=π/2,β= 2π/3, (d)θ~0,β=0, and (e)θ=π/14,β= 0 ~ 2π. The bottom panel shows the raster scanning TPF images of five patterns retrieved at corresponding polarization orientations. Scale bar, 10 μm. Figure 4: Demonstration of 3D orientation-unlimited polarization encryption. The red arrows in ( a–e ) indicate the five configured polarization orientations used for the information encryption at ( a ) θ = π /2, β = 0, ( b ) θ = π /2, β = π /3, ( c ) θ = π /2, β = 2 π /3, ( d ) θ ~0, β =0, and ( e ) θ = π /14, β = 0 ~ 2 π . The bottom panel shows the raster scanning TPF images of five patterns retrieved at corresponding polarization orientations. Scale bar, 10 μm. Full size image We have demonstrated the arbitrary 3D control of the focal polarization orientation by using a single optically configured vectorial beam. This is achieved by the superposition of radially and azimuthally polarized beams, diffracted by a high NA objective. Parametrically configuring the input polarization state has led to the demonstration of the orientation-unlimited polarization states in the focus as well as its application in polarization information encryption. Consequently, this orientation-unlimited flexibility enables polarization encryption with a 3D arbitrary 'key' polarization-generation capability, therefore facilitating an ultra-security protocol. In addition, the demonstrated technique paves the way for polarization microscopy to tailor the light-matter interaction in an orientation-unlimited 3D manner, for example, for single molecule detection, multi-dimensional optical data storage, 3D display and spintronics. Orientation-unlimited 3D polarization Two twisted nematic liquid crystal devices (Arcoptix S. A.) [23] were inserted in the beam paths to convert the linear polarization into radially and azimuthally polarized beams, respectively. The amplitude apodizer is either a concentric obstruction disc with a normalized radius or an off-centre open aperture with azimuthally variable transmission given by |cos( φ − α )|, where φ and α are the azimuthal angle and the transmission axis of off-centre disc, respectively ( Supplementary Fig. S1 ). The vectorial beam at the back aperture of the objective can be written as the superposition of radial and azimuthal beams E = P ( α , )( γ · e r + δ · e φ ), where P ( α , ) is the pupil apodization function of the apodizer, e r and e φ are the unit vectors in the radial and azimuthal directions, respectively. The focal field of the superposed vectorial beam can be derived by the vectorial diffraction theory as [13] , [16] where A is a constant, u is the convergence angle, a is the maximum angle of convergence determined by the numerical aperture of the objective, J n ( x ) is the n th order Bessel function of its first kind and φ is the azimuthal angle in the image plane. The ratio of the averaged longitudinal to transverse polarization intensity components within the focal plane defined by the full width at half maximum (FWHM) can be expressed as Although the ratio of the polarization field components is generally used to define the polarization angle at individual points in free space, the ratio of the energy between different polarization components averaged within the focal plane is more relevant when the threshold effect of material response is considered during the polarized light interaction with materials, for example, in the polarization encryption with nanorods. Therefore, we define the out-of-plane orientation angle of the resultant polarization as Configuring the weighting factor tan −1 ( δ / γ ) and the radius of the concentric obstruction disc of the apodizer P (α=0, ) of the single vectorial beam can arbitrarily adjust the ratio of the longitudinal to transverse polarization field and intensity components, respectively ( Supplementary Fig. S2 ). Fluorescence rate calculation The raster scanning TPF image of a single gold nanorod located at a given position r represents the fluorescence-rate distribution, which is given by [19] R ( r )= c | d . E ( r )| 4 , where d is the unit vector of the absorption dipole aligned along the nanorod orientation, and E ( r ) is the electric field of the excitation beam at the position of the single nanorod and c is a constant. Optical microscope set-up Both TPF scanning and polarization encryption were conducted in the same homebuilt microscope. To excite TPF, a femtosecond-pulsed laser (SpectraPhysics Tsunami, 100 fs pulse duration and 80 MHz repetition rate), at 780 nm wavelength, was employed. The fluorescence was detected in the 400–700 nm wavelength range by a Hamamatsu PMT (H7422-40P). The TPF contrast is defined as ( I − I bg )/( I + I bg ), where I and I bg are the TPF signals of the nanorods and the background, respectively. For polarization encryption, an electro-optic modulator was used to gate pulses from the pulse train. Sample preparation Gold nanorods with an extinction peak at the wavelength of 790 nm and an average aspect ratio of 4.0±1 were prepared following the wet chemical methods [24] . The diluted nanorods solution with an optical density of 0.25 was drop-casted on the polyvinyl alcohol-coated cover glass to enrich the 3D random distribution while well separated to prevent aggregation. To prepare the gold nanorod mixed polymer sample for polarization encryption, the gold nanorod solution with an optical density of 100 mixed with a 15 wt% polyvinyl alcohol solution was drop-casted and dried on a cover glass. The approximate nanorod concentration in the film was 500±50 nM (ref. 25 ). Optimizing the repetition rate of pulsed laser excitation Although the excitation and melting of gold nanorods can be sharply selected by configuring the 3D polarization orientation, the unselected gold nanorods could still be affected or damaged by accumulative temperature rise of the embedded matrix, polyvinyl alcohol, as a result of the high repetition rate of the pulsed laser beam [20] , [22] . An electro-optic modulator was used to gate pulses from the pulse train of repetition rate 80 MHz to 100 kHz and 1 kHz. No pronounced difference was observed once the repetition rate is below 1 kHz, because the inter-pulse separation is 1 ms, which is significantly longer than the heat diffusion time of microseconds [26] for the given focal region. The comparison of the averaged contrast of the 16 patterned bits normalized to that of the voids, as a result of deformation of the matrix, clearly revealed that the pulse energy that the sample can stand, or the dynamic range, is much broader at 1 kHz than that at higher repetition rates of 100 kHz and 80 MHz. In other words, at the 1 kHz repetition rate, the polarization unselected gold nanorods remain unaffected during the 3D polarization encryption ( Supplementary Fig. S4 ). How to cite this article: Li, X. et al . Three-dimensional orientation-unlimited polarization encryption by a single optically configured vectorial beam. Nat. Commun. 3:998 doi: 10.1038/ncomms2006 (2012).